Integrated exome and transcriptome sequencing revealsZAKisoform usage in gastric cancer Gastric cancer is the second leading cause of worldwide cancer mortality, yet the underlying genomic alterations remain poorly understood. Here we perform exome and transcriptome sequencing and SNP array assays to characterize 51 primary gastric tumours and 32 cell lines. Meta-analysis of exome data and previously published data sets reveals 24 significantly mutated genes in microsatellite stable (MSS) tumours and 16 in microsatellite instable (MSI) tumours. Over half the patients in our collection could potentially benefit from targeted therapies. We identify 55 splice site mutations accompanied by aberrant splicing products, in addition to mutation-independent differential isoform usage in tumours. ZAK kinase isoform TV1 is preferentially upregulated in gastric tumours and cell lines relative to normal samples. This pattern is also observed in colorectal, bladder and breast cancers. Overexpression of this particular isoform activates multiple cancer-related transcription factor reporters, while depletion of ZAK in gastric cell lines inhibits proliferation. These results reveal the spectrum of genomic and transcriptomic alterations in gastric cancer, and identify isoform-specific oncogenic properties of ZAK. Gastric cancer is the fourth most common cancer and the second most common cause of cancer-related death worldwide [1] . While several chemotherapy options are available for treating gastric cancer patients, the only available targeted therapy choice is trastuzumab for ERBB2-positive patients [2] . The heterogeneous nature of gastric cancer and the lack of targeted therapy options present an urgent need for detailed understanding of genomic alterations in gastric cancer, as such characterization can suggest therapeutic targets and patient stratification strategies. Previous exome sequencing of 15–22 gastric tumours identified TP53 and ARID1A as frequently mutated genes [3] , [4] , but there was only limited overlap of most significantly mutated genes between these studies [5] , suggesting that more in-depth genomic characterization of gastric cancer is needed. In addition, transcriptome sequencing coupled with genomic analysis has not been performed for gastric cancer, thus it has been difficult to investigate how the reported mutations are related to transcriptional changes. Cancer-specific splicing isoforms, in particular, represent an important class of gene product for executing distinct biochemical functions. Cancer-specific splicing products can result from both differential expression and regulation of splicing factors and somatic mutations impacting critical splicing signals, but the prevalence of such events is not known. Regardless of the underlying mechanisms, the identification of cancer-specific splicing products could broaden the search space for cancer-causing proteins. This is especially relevant to gastric cancer, since currently known coding-region mutations can explain the genetic basis in only a small fraction of the patients [3] , [4] , [5] . Here we apply whole-exome sequencing, RNA sequencing and single nucleotide polymorphism (SNP) array technology to characterize 51 human primary gastric tumour and adjacent normal samples, and 32 gastric cancer cell lines ( Supplementary Data 1–3 ). We examine the somatic mutation spectrum with respect to the microsatellite stability status, and aim to identify mutations or DNA copy number changes that might suggest clinical treatment options. We then focus on combining the RNA- and DNA-level information to identify both mutation-dependent aberrant splicing and mutation-independent splicing isoforms in gastric cancer. We further identify an isoform of the ZAK kinase that is specifically implicated in gastric cancer. Viral and bacterial pathogens are known to play a role in the development of gastric cancer [6] . Therefore, we first conducted transcriptome analysis to identify pathogen sequences in gastric samples. Notably, five of the tumours but none of the normal samples had Epstein-Barr virus ( Human herpesvirus 4 ) sequences ( Supplementary Figs 1 and 2 ), although the enrichment does not reach statistical significance due to small sample size ( N =80, P =0.06, Fisher’s exact test). Sequences of Helicobacter pylori , known to be associated with gastritis and gastric cancer [6] , were found in most samples and not significantly enriched in tumours ( Supplementary Fig. 1 ). We identified a total of 27,732 somatic mutations in our exome data from 48 tumour-normal sample pairs. Forty per cent (11,112) were protein-altering (8,726 missense, 1,661 indels, 494 nonsense, 10 stop loss and 221 essential splice site. Supplementary Data 4–6 ). MSI is an aetiological source of somatic mutations and is observed in 10–30% of gastric tumours [7] . Consistent with previous findings [3] , the 10 MSI tumours in our collection harboured many more protein-altering mutations than the 38 MSS samples (median: 643 for MSI versus 83 for MSS, N =48, P =2 × 10 −6 , one-tailed Wilcoxon rank sum test, Fig. 1a ). The difference was especially pronounced for insertions and deletions, with MSI samples containing ~90 times more indels than MSS (median: 132 for MSI versus 1.5 for MSS, N =48, P =6 × 10 −7 , one-tailed Wilcoxon rank sum test, Fig. 1a ). Notably, all five tumour samples with Epstein-Barr virus RNAseq reads were MSS, and those samples had more mutations than other MSS samples ( N =37, P =0.01, one-tailed Wilcoxon rank sum test). In our data set, we identified 30 recurrent somatic mutations in tumours ( Supplementary Data 7 ). In total, 94 (1%) of the protein-altering somatic variations identified in this study have been reported in at least two unique samples in the Catalogue of Somatic Mutations in Cancer [8] ( Supplementary Data 4 ), suggesting that they may be driver mutations. 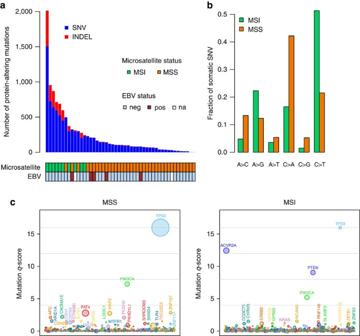Figure 1: Somatic mutations in gastric cancer. (a) Number of somatic protein-altering mutations per tumour. Epstein-Barr virus (EBV) status (according to the presence of EBV reads in RNAseq data) and microsatellite status are shown below. EBV status for two samples is not available due to the absence of RNAseq data for the samples. (b) Mutation spectrum varies between MSI and MSS samples. (c) Recurrently mutated genes for MSS (left) and MSI (right) samples by MuSiC analysis. Each circle represents a gene and the size of the circle is proportional to the mutation count for that gene. The genes are represented in alphabetical order from left to right on thexaxis. Genes with a statistically significantq-value are labelled. Figure 1: Somatic mutations in gastric cancer. ( a ) Number of somatic protein-altering mutations per tumour. Epstein-Barr virus (EBV) status (according to the presence of EBV reads in RNAseq data) and microsatellite status are shown below. EBV status for two samples is not available due to the absence of RNAseq data for the samples. ( b ) Mutation spectrum varies between MSI and MSS samples. ( c ) Recurrently mutated genes for MSS (left) and MSI (right) samples by MuSiC analysis. Each circle represents a gene and the size of the circle is proportional to the mutation count for that gene. The genes are represented in alphabetical order from left to right on the x axis. Genes with a statistically significant q -value are labelled. Full size image Analysis of the base-level mutation spectrum showed that C-to-A transversions were most common in MSS samples (42%), while C-to-T transitions predominated in MSI tumours (51%) ( Fig. 1b ). The increase in C-to-T transitions in MSI samples is consistent with the results from a DNA mismatch repair-deficient mouse model [9] . Sequence analysis of the flanking nucleotides revealed an enrichment of G following the C-to-T transitions in both MSS and MSI samples ( Supplementary Fig. 3 ). To identify significantly mutated genes, we combined our data with the previously published gastric exome data sets [3] , [4] , and applied the MuSiC [10] algorithm to MSI and MSS samples separately. The meta-analysis of three data sets not only confirmed recurrent mutated genes highlighted in previous gastric exome studies, such as ARID1A [3] and FAT4 (ref. 4 ), but also greatly increased our statistical power to detect significantly mutated genes. TP53 and PIK3CA were the only genes found to be significant in both MSI and MSS samples ( Fig. 1c and Supplementary Data 8 ). Other significantly mutated genes in MSS samples included some of the known cancer drivers, such as ARID1A , APC , CTNNB1 , CDH1 and SMAD4 . In addition, we identified a few genes not previously implicated in gastric cancer: putative tumour suppressor proteins LDOC1 (refs 11 , 12 ) and PCDH9 (ref. 13 ), and cell surface proteins ELTD1 , GPC6 , TLR4 and PKHD1L1 . In MSI samples, we identified 16 significantly mutated genes, including known oncogenes KRAS and ERBB2 . Other potential novel driver candidates include ZBTB1 , TRAPPC2L , as well as G protein-coupled receptors GPR39 , GPR85 and CHRM3. Notably, in our gastric cell line collection we also observed 17 protein-altering point mutations or indels in TP53 , 14 in APC , 12 in FAT4 , 8 in CDH1 and 5 in PIK3CA ( Supplementary Data 9 and 10 ). We further examined genes affected by either protein-altering mutations or substantial copy number alterations in our tumour samples ( Supplementary Fig. 4 , Supplementary Note 1 , Supplementary Data 11 and 12 ), and aggregated them into defined and curated pathways that are known to be involved in cancer [14] by constructing a pathway aberration incidence matrix. Among the highly altered pathways were several known cancer pathways such as TP53, RTK, PI3K and cell cycle ( Fig. 2a ). Notably, alteration of the PI3K pathway is significantly associated with the MSI group ( N =43, Benjamini–Hochberg-adjusted P -value=0.007, Fisher’s exact test): 9/10 MSI samples have alterations in the pathway, compared with only 8/33 for MSS samples ( Fig. 2b ). In addition, very few copy number changes contributed to pathway alterations in the MSI samples ( Fig. 2b ), confirming that point mutations drive oncogenic deregulation in these samples. 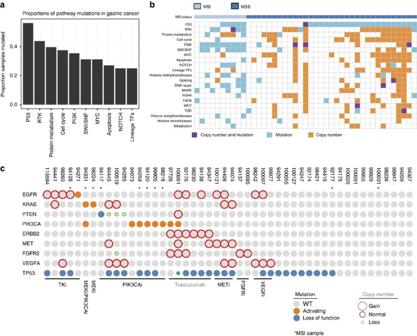Figure 2: Altered pathways in gastric cancer and potential targeted therapies. (a) Barplot showing the fraction of samples containing an aberration in curated pathways. Top 10 most altered pathways are shown. Aberrations are defined as mutations or copy number changes in any of the pathway member genes. (b) Matrix showing the distribution of pathway aberrations per sample ordered from most frequently aberrant pathway (top) to least frequently aberrant pathway (bottom). Colours of the matrix indicate whether the pathway was affected by mutation (blue), copy number change (magenta) or both (orange). The colour bar on top shows MSI (green) or MSS (orange) status. (c) Potential targeted therapies that can be applied to this patient population, based on the status of amplification, known activating mutations or loss-of-function mutations of key cancer genes. Figure 2: Altered pathways in gastric cancer and potential targeted therapies. ( a ) Barplot showing the fraction of samples containing an aberration in curated pathways. Top 10 most altered pathways are shown. Aberrations are defined as mutations or copy number changes in any of the pathway member genes. ( b ) Matrix showing the distribution of pathway aberrations per sample ordered from most frequently aberrant pathway (top) to least frequently aberrant pathway (bottom). Colours of the matrix indicate whether the pathway was affected by mutation (blue), copy number change (magenta) or both (orange). The colour bar on top shows MSI (green) or MSS (orange) status. ( c ) Potential targeted therapies that can be applied to this patient population, based on the status of amplification, known activating mutations or loss-of-function mutations of key cancer genes. Full size image Currently, the only approved targeted therapy for gastric cancer is trastuzumab for ERBB2 -positive tumours. Several others in clinical trials or approved for other indications include EGFR inhibitors, MEK inhibitors for KRAS -mutant tumours, PIK3CA and MET inhibitors (phase III, gastric cancer). When we examined alterations in these genes, we identified six samples with ERBB2 amplification and five harbouring MET amplification ( Fig. 2c ). In addition, we found several known activating mutations, including two KRAS -activating mutations, 8 PIK3CA -activating mutations and one EGFR -activating mutation (out of 4 EGFR mutations in our samples). Collectively, more than half of the patients in our sample set harbour activating alterations in targetable genes and would potentially benefit from therapies that are approved or in clinical trials ( Fig. 2c ). Furthermore, we identified six patients with ERBB2 point mutations including a recurrent R678Q change ( Supplementary Data 4 ). None of these match with the activating ERBB2 point mutations recently identified in breast tumours [15] , so it remains unclear whether gastric cancer patients with ERBB2 mutations would benefit from the trastuzumab treatment. The combined exome and RNAseq data enable global analysis of mutations potentially affecting mRNA splicing. We identified 139 mutations affecting essential splice donor or acceptor sites of genes that have RNA splice junction reads spanning the splice site mutations. Among those mutations, 80 had spanning junctions that were not consistent with annotated exon models. By further excluding junctions present in any normal gastric tissue samples, we obtained a list of 55 mutations that are associated with tumour-specific aberrant splice junctions ( Supplementary Fig. 5a and Supplementary Data 13 ). Thus, about 40% (55/139) of essential splice site mutations showed evidence of altered splicing. Since these mutations were heterozygous, we typically observed both known and aberrant splice junctions spanning the same mutation locus; the number of reads supporting normal junctions was much higher than those supporting aberrant junctions ( Supplementary Fig. 5b ), possibly due to nonsense-mediated decay of the aberrant transcripts. Several of the 55 genes with evidence of aberrant splicing were known cancer-related genes including TP53 , MAP2K4 (JNKK) and CHD8 ( Supplementary Data 13 ; Supplementary Fig. 6 ). Mutations in MAP2K4 were previously found in a variety of human malignancies [8] , [16] , [17] , [18] , including gastric cancer cell lines [18] ( Supplementary Fig. 7 ). We found 4 mutations in MAP2K4 in our tumour collection, including one missense, two splice site and one frameshift. In tumour sample SAM94128, where we identified a mutation affecting the AG splice acceptor sequence ( Supplementary Fig. 6a ), the RNAseq data showed eight reads supporting the expression of a novel isoform of MAP2K4 that skips exon 8, leading to an in-frame deletion of 26 residues, thereby disrupting the essential protein kinase domain. The loss-of-function nature of the mutation is consistent with the suggested tumour suppressor role of MAP2K4 (refs 17 , 18 ). We performed differential expression analysis on the transcriptome sequencing data. The expression level and variability of smoothelin (a smooth muscle expression marker (SMTN)) was significantly higher in our normal gastric tissue samples than gastric tumours ( Supplementary Fig. 8a , left panel), indicating varying degree of smooth muscle contamination in the normal tissues. After including the SMTN term in our statistical model to account for the contamination effect, we found 165 upregulated and 256 downregulated genes in tumours using a stringent cutoff (fold change >3 and Benjamini–Hochberg adjusted P -value <10 −10 ) ( Supplementary Note 2 and Supplementary Data 14 ). These include many canonical markers for gastric cancer like serum markers MUC5AC [19] , Reprimo [20] and Pepsinogen C [21] . A significant proportion of the 165 genes with higher expression in tumours are involved in cell cycle ( P =10 −6 ), while digestion, transmembrane transport and ion transport functions were downregulated. We also found 22 gene fusions ( Supplementary Note 3 , Supplementary Data 15 and Supplementary Fig. 9 ), but detailed analysis of these fusions did not support a driver role for any of them. The transcriptome data also allowed us to identify splice isoforms related to cancer. Isoform usage was quantified by tallying the reads uniquely assignable to a particular isoform, and then comparing those to reads mapped to the entire gene (that is, all known isoforms). The significance of differential isoform usage was assessed by a generalized mixed-effect regression model using negative binomial as the underlying model. After correcting for the smooth muscle contamination, we identified 170 genes with differential isoform usage between tumours and paired normal tissue. These included cancer-related genes such as ZAK , KRAS , MCM7 , ELK4 and CCND3 ( Supplementary Data 16 ). We focused our attention on ZAK (sterile alpha motif and leucine zipper containing kinase AZK, also known as MLTK ) because it exhibited one of the smallest P -values among the cancer-related kinases, a major cancer target class. ZAK is a component of stress-activated signal transduction cascade, which has been implicated in several pathways related to cancer, such as apoptosis, cell cycle and neoplastic cell transformation [22] , [23] , [24] . ZAK has two major transcript variants TV1 and TV2. Protein products of TV1 (MLTK-α) and TV2 (MLTK-β) share the same N terminus that contains a kinase domain. TV1 has a longer C-terminal region containing a sterile alpha motif; while TV2 has a conserved unique C-terminal extension of 124 amino acids including an extended acidic patch ( Fig. 3a ). Previous studies suggest that the two isoforms of ZAK may have distinct biological functions, with TV1 being specifically implicated in histone phosphorylation [25] and disruption of actin stress fibres [26] . 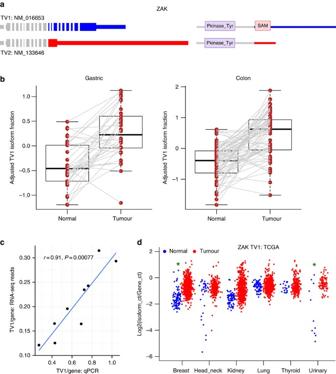Figure 3: Differential ZAK isoform usage between normal and tumour samples. (a)ZAKgene model and protein domain structure. Thick bars: coding exons; thin bars: UTR. TV2 lacks the last nine exons and has a long terminal coding and non-coding exon. Blue and red indicate unique TV1 and TV2 sequences. Transcript variant 1 (TV1) encodes a longer protein product with a sterile alpha motif domain. (b) ZAK TV1 fraction is significantly higher in gastric tumours (left) and colon tumours (right), compared with normal adjacent tissues. The fraction of TV1 was measured by the ratio between the number of reads uniquely assignable to TV1 and the number of reads mapped to the entireZAKgene. To account for smooth muscle contamination in normal tissues, we fit a linear model with smoothelin expression as predictor and the log isoform fraction as response, and used the residuals of the model as the ‘adjusted isoform fraction’. Dots represent samples. Grey lines connect matched tumour and normal samples. The boxes in the box-and-whisker plots represent the interquartile range between the first and third quartiles; the dashed lines (whiskers) extend to the most extreme data points, which is no more than 1.5 times the interquartile range from the box. (c) ZAK isoform fractions derived from RNAseq data correlate with quantitative PCR (qPCR) measurements. For nine gastric cancer cell lines in our study, we quantified the ratio between ZAK total expression and ZAK TV1 expression using qPCR, and compared the measurements with the isoform fraction we derived from the RNAseq data. The two measurements have significant correlation (Pearson’s correlation coefficientr=0.91,P-value=0.00077). (d) ZAK isoform expression in six TCGA data sets where there are >10 normal samples. Normal samples are represented by blue dots and tumour samples by red dots. ZAK TV1 fraction is significantly higher (adjustedP-value <0.001 and fold change >2) in breast and bladder cancer data (marked by the green asterisks). Figure 3: Differential ZAK isoform usage between normal and tumour samples. ( a ) ZAK gene model and protein domain structure. Thick bars: coding exons; thin bars: UTR. TV2 lacks the last nine exons and has a long terminal coding and non-coding exon. Blue and red indicate unique TV1 and TV2 sequences. Transcript variant 1 (TV1) encodes a longer protein product with a sterile alpha motif domain. ( b ) ZAK TV1 fraction is significantly higher in gastric tumours (left) and colon tumours (right), compared with normal adjacent tissues. The fraction of TV1 was measured by the ratio between the number of reads uniquely assignable to TV1 and the number of reads mapped to the entire ZAK gene. To account for smooth muscle contamination in normal tissues, we fit a linear model with smoothelin expression as predictor and the log isoform fraction as response, and used the residuals of the model as the ‘adjusted isoform fraction’. Dots represent samples. Grey lines connect matched tumour and normal samples. The boxes in the box-and-whisker plots represent the interquartile range between the first and third quartiles; the dashed lines (whiskers) extend to the most extreme data points, which is no more than 1.5 times the interquartile range from the box. ( c ) ZAK isoform fractions derived from RNAseq data correlate with quantitative PCR (qPCR) measurements. For nine gastric cancer cell lines in our study, we quantified the ratio between ZAK total expression and ZAK TV1 expression using qPCR, and compared the measurements with the isoform fraction we derived from the RNAseq data. The two measurements have significant correlation (Pearson’s correlation coefficient r =0.91, P -value=0.00077). ( d ) ZAK isoform expression in six TCGA data sets where there are >10 normal samples. Normal samples are represented by blue dots and tumour samples by red dots. ZAK TV1 fraction is significantly higher (adjusted P -value <0.001 and fold change >2) in breast and bladder cancer data (marked by the green asterisks). Full size image We observed significant increase in the fraction of ZAK TV1, indicating preferential upregulation of TV1 in tumours ( Fig. 3b , left panel, P =1.4 × 10 −9 , see Methods for detailed description of statistical analysis). The quantification of isoform fractions from our RNAseq data was supported by quantitative PCR measurements ( Fig. 3c ). We also used Cufflinks as an alternative method for transcript isoform quantification and confirmed that TV1 expression was higher in the tumours than in the normals, while TV2 expression remained unchanged ( Supplementary Fig. 8b ). To analyse isoform-specific ZAK expression in situ , we performed in situ hybridization using probes specific to the different ZAK isoforms ( Supplementary Methods ). Consistent with the transcriptomic analysis, ZAK TV1 expression was found upregulated in gastric cancer, while TV2 was more ubiquitously expressed in gastric tumour cells as well as normal mucosa and smooth muscle ( Supplementary Fig. 10 ). The preferential upregulation of ZAK TV1 is seen in several other cancers. Analysis of colorectal cancer RNAseq data [27] showed that the fraction of TV1 increased by about threefold ( P <10 −20 , Fig. 3b , right panel), and ZAK was reported to be one of the top candidate genes to modulate β-catenin-dependent transcription and regulate colon cancer cell proliferation in two loss-of-function screens [28] . The Cancer Genome Atlas (TCGA) RNAseq data also showed significantly higher ZAK TV1 usage in bladder and breast cancer relative to corresponding normal samples ( Fig. 3d ). We only detected one non-synonymous mutation and one frameshift insertion in ZAK in our tumour samples and one additional point mutation in the cell lines, suggesting that expression of ZAK isoforms in these samples may be regulated by trans-acting splice factors instead of mutations in the ZAK gene itself. To validate our findings from RNAseq and characterize ZAK activity in gastric cancer, we tested ZAK function in gastric cancer cell lines. ZAK TV1 protein was upregulated in gastric tumours and cell lines relative to normal stomach ( Fig. 4a ). Overexpression of TV1, but not of TV2, induced robust transcriptional activation of several cancer-related signalling genes such as AP1 and NFkB , known to be modulated by ZAK activity [22] ( Fig. 4b ). Depletion of ZAK using two independent short hairpin RNAs (shRNAs) led to significant growth inhibition in gastric cell lines that express high levels of ZAK TV1 and variable levels of TV2 ( Fig. 4c ). These observations suggest an important role for ZAK TV1 in activating cancer signalling pathways and gastric cancer growth. 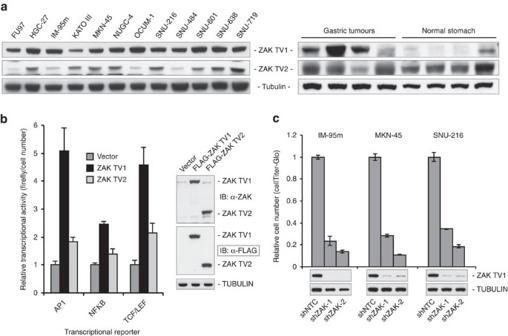Figure 4: Experimental validation of ZAK function in cancer. (a) Immunoblots of ZAK TV1 and TV2 expressions show that protein level of TV1 is higher in gastric tumours and cell lines, compared with normal stomach tissues. ZAK TV1 was detected with Bethyl α-ZAK antibody and TV2 with Sigma α-ZAK antibody (see Methods). (b) ZAK TV1, but not TV2, can stimulate multiple transcriptional programs related to cancer pathways. Transcription reporter assay in 293 cells transfected with empty vector, TV1 or TV2 along with the indicated firefly luciferase reporter construct (AP1, NFkB and TCF/LEF). Activity is normalized to cell number using CellTiter-Glo. Immunoblot shows relativeZAKisoform expression from 293 cells transfected with the indicated construct. ZAK was detected with Sigma α-ZAK antibody. (c) Depletion ofZAKfrom gastric cancer cell lines inhibits cell growth. In cell lines where ZAK knockdown led to reduced viability, there was consistently high TV1 expression, while TV2 expression was marginal and variable (for example, IM-95m cell line, see for example, panela). Cell viability analysis was carried out 6 days after infection of gastric cancer cell lines with independentZAKshRNAs. Cell number is normalized to shNTC-infected cells. Immunoblot indicates the level of ZAK-TV1 depletion 4 days after infection. ZAK was detected with Bethyl α-ZAK antibody. Figure 4: Experimental validation of ZAK function in cancer. ( a ) Immunoblots of ZAK TV1 and TV2 expressions show that protein level of TV1 is higher in gastric tumours and cell lines, compared with normal stomach tissues. ZAK TV1 was detected with Bethyl α-ZAK antibody and TV2 with Sigma α-ZAK antibody (see Methods). ( b ) ZAK TV1, but not TV2, can stimulate multiple transcriptional programs related to cancer pathways. Transcription reporter assay in 293 cells transfected with empty vector, TV1 or TV2 along with the indicated firefly luciferase reporter construct (AP1, NFkB and TCF/LEF). Activity is normalized to cell number using CellTiter-Glo. Immunoblot shows relative ZAK isoform expression from 293 cells transfected with the indicated construct. ZAK was detected with Sigma α-ZAK antibody. ( c ) Depletion of ZAK from gastric cancer cell lines inhibits cell growth. In cell lines where ZAK knockdown led to reduced viability, there was consistently high TV1 expression, while TV2 expression was marginal and variable (for example, IM-95m cell line, see for example, panel a ). Cell viability analysis was carried out 6 days after infection of gastric cancer cell lines with independent ZAK shRNAs. Cell number is normalized to shNTC-infected cells. Immunoblot indicates the level of ZAK-TV1 depletion 4 days after infection. ZAK was detected with Bethyl α-ZAK antibody. Full size image This study represents the largest integrated genomic and transcriptomic analysis of gastric cancer to date. Our meta-analysis of three gastric exome data sets provides the most comprehensive characterization of the recurrently mutated genes in gastric cancer. We also identified 170 genes with distinct isoform usage patterns between tumour and normal samples. In particular, the ZAK TV1 isoform is preferentially upregulated in gastric tumours and cell lines, resulting in significantly higher TV1 fraction. This pattern was seen in several other cancer types, suggesting a widespread association of ZAK TV1 with tumorigenesis. Recently, ZAK TV1, but not TV2, has been shown to stimulate anchorage-independent colony growth and xenograft tumour formation [29] , further supporting the oncogenic role of this particular isoform. These cancer-specific isoforms can dramatically broaden opportunities in cancer classification and tumour-specific anti-cancer targets. Sample preparation We characterized primary tissue samples from 51 gastric cancer patients ( Supplementary Data 1 ) and 32 gastric cancer cell lines ( Supplementary Data 2 ). Fresh-frozen primary gastric tumours and adjacent normal tissue samples were obtained from SeraCare LifeSciences, ILSBio, ProteoGenex, University of Michigan, and Cureline, Inc. All samples used in the study had approval from institutional review board and informed consent from study participants. All tumour and normal tissues were subjected to pathology review to confirm diagnosis and tumour content. Only tumours with >50% tumour content and their corresponding matched normal tissues (if available) were included in this study. The Qiagen AllPrep DNA/RNA kit was used to prepare DNA and RNA. Tumour samples were assessed for MIS using an MSI detection kit (Promega). Gastric cancer cell lines were obtained from DSMZ, KCLB, JCRB, ECACC, ATCC, Riken and Teva ( Supplementary Data 2 ). High-throughput sequencing of exomes and transcriptomes Exome capture was performed using the Nimblegen SeqCap EZ Human Exome Library v2 (44 Mb) or Agilent SureSelect Human All Exome kit (50 Mb). Exome capture libraries were sequenced by HiSeq 2000 (Illumina) to generate 2 × 75 bp paired-end data ( Supplementary Data 3 ). We also obtained RNAseq data using the TruSeq RNA Sample Preparation kit (Illumina). Libraries were multiplexed two per lane and sequenced on HiSeq 2000 to obtain at least 30 million paired-end (2 × 75 bp) reads per sample. All sequencing reads were evaluated for quality using the Bioconductor ShortRead package. Sample identity was confirmed by comparing genotype data derived from exome sequencing and RNAseq against Illumina 2.5 M array data. Samples derived from the same patient were expected to have >80% concordance. Samples failing the criteria were excluded. Variant calling and validation Sequence reads were mapped to the UCSC human reference genome (GRCh37/hg19) using Burrows-Wheeler Aligner software [30] with default parameters. Local realignment and duplicate removal were performed as described [31] . Somatic mutations were determined for each sample from the corresponding tumour and matched normal BAM files using Strelka [32] . Strelka variants were additionally filtered to include only variants with a minimum variant quality of 30, a minimum variant allele frequency of 5% and a variant allele frequency in the matched normal of <5%. Known germline variations seen in dbSNP Build 131 (ref. 33 ) or 6,515 normal exomes [34] but not in COSMIC v56 (ref. 8 ) were excluded. For cell lines, variants were determined using the GATK UnifiedGenotyper [31] . Known germline variants were screened out if it they were not represented in COSMIC in at least two samples and were present in one of the following data sources: dbSNP Build 131 (ref. 33 ), 6,515 previously published normal exomes [34] , germline variants from this study and germline variants from previous publications [27] , [35] . Mutational significance We evaluated the mutational significance of genes using MuSiC [10] for both the MSI and MSS samples separately given their different background mutation rates. Genes with very low expression (RPKM<0.17, the lower quartile among expressed genes) were excluded from this analysis. Q scores were calculated by taking the negative log10 of the FDR CT values from MuSiC with a maximum possible value of 16. Analysis of pathway aberration We aggregated genomic mutations and copy number changes into defined and curated pathways that are known to be involved in cancer [14] by constructing a binary pathway aberration matrix. For each sample we called a pathway aberrant if any of the genes in the pathway contained a somatic mutation or a significant copy number change in that sample. Significant copy number changes were either amplifications (median centred, ploidy-corrected copy number >0.3) or losses (median centred, ploidy-corrected copy number <−0.4). Somatic mutations were limited to mutations that caused a premature stop codon, were previously annotated in COSMIC [8] or were predicted to be deleterious by the Condel algorithm [36] . RNAseq data processing and expression analysis RNAseq reads were first aligned to ribosomal RNA sequences to remove ribosomal reads. The remaining reads were aligned to the human reference genome (NCBI Build 37) using GSNAP [37] version ‘2012-01-11’, allowing maximum of two mismatches per 75 base sequence (parameters: ‘-M 2 -n 10 -B 2 -i 1 -N 1 -w 200000 -E 1 --pairmax-rna=200,000’). Transcript annotation was based on the RefSeq database downloaded on 30 November 2011. To quantify gene expression levels, the number of reads mapped to the exons of each RefSeq gene was calculated. Differential expression analysis on the count data was performed using the R package ‘DESeq2’ [38] , which is based on a negative binomial distribution and uses shrinkage estimation for the variance of the distribution. As an alternative way of quantifying normalized gene and transcript expression, Fragments Per Kilobase of transcript per Million mapped reads (FPKM) values were also derived using Cufflinks [39] (version 2.1.1). Raw data of TCGA cancer RNAseq data sets were downloaded from the TCGA repository ( http://cancergenome.nih.gov/ ) and processed in the same way as our in-house data. Essential splice site mutations and aberrant splicing events Somatic mutations at essential splice sites (the first and last two bases of introns) were extracted from the list of somatic mutations in 32 tumours with both exome and RNAseq data. Splice junction reads spanning the splice site mutations were extracted from the RNAseq data. To more stringently define aberrant splice junctions, we checked the splice junction reads against transcript models from both RefSeq and UCSC, and only those junctions inconsistent with both sources were called aberrant. Differential isoform usage between cancer and normal samples Total read counts for each gene, as well as counts of reads that can be uniquely assigned to a particular isoform, were obtained from the BAM files. Differential isoform usage was assessed on isoforms with sufficiently high number of counts using a negative binomial regression model. Specifically, for each gene we calculated the 75th percentile of gene read counts in tumour samples and, separately, in normal samples. Any gene with the 75th percentile below 20 in either set of samples were excluded from further analysis. Similarly, for each isoform we calculated 75th percentile of isoform-specific read counts in two sets of samples and excluded isoforms with 75th percentile below 10. We then fit a generalized mixed-effect negative binomial regression model to isoform-specific read counts, using tumour/normal status (fixed effect) and patient identifier (random effect) as main covariates and gene-level read counts as offset. Since we observed variable smooth muscle inclusion in our normal tissue samples, we also included the expression of smoothelin (SMTN) in our model to correct for the extent of the smooth muscle inclusion. The model was fit using the ‘glmer.nb’ function in the ‘lme4’ R package [40] independently for each isoform as follows: glmer.nb(Isoform.ct~TumorStatus+(1|Patient)+log(SMTN)+offset(log(Gene.ct))). The reported P -values corresponding to TumorStatus coefficient estimates for each isoform were adjusted using Bonferroni correction. Transcript isoforms with significantly differential isoform usage (adjusted P -value <0.1 and fold change >1.5) were selected for further investigation. To visualize the differential isoform usage, we fit a linear model lm(log2(Isoform.ct/Gene.ct)~log(SMTN)), and used the residuals of the model as the ‘adjusted isoform fraction’ for individual samples. To further narrow down the list of candidate genes for experimental validation, we focused on cancer-related genes. Genes are defined as cancer related if they appear in either Cancer Gene Census [41] or cancer-related canonical pathways in Molecular Signatures Database [42] (v3.0), including AKT, cell cycle, death receptor signalling, ERBB, ERK, MAPK, MTOR, NFkB, Notch, P53, PTEN, VEGF and WNT pathways. To assess the accuracy of our method, we performed systematic simulations. The detailed procedure and results of our simulation are presented in Supplementary Methods and Supplementary Fig. 11 . Expression quantification by TaqMan assays The TaqMan probe and primer assays for ZAK (Hs00370448_m1 for entire gene, Hs00928997_m1 for TV1) and glyceraldehyde 3-phosphate dehydrogenase (GAPDH Hs00266705_g1) were obtained from Life Technologies, CA. RNA was isolated from cells using TRIzol (Invitrogen, CA). Gene and isoform expression was measured using the Quantitect Probe RT-PCR kit (Qiagen, CA, kit# 204443) with 50 ng of RNA and appropriate probe primer set. The samples were first held at 50 °C for 30 min for reverse transcription, and then at 95 °C for 15 min. This was followed by 40 cycles at 94 °C for 15 s and 60 °C for 1 min on an ABI ViiA7 Sequence Detection System (Life Technologies). Data were analysed using Δ C t method by normalizing to GAPDH. The TaqMan reactions were performed in duplicates to obtain the mean values. Cell lines and culture conditions The gastric cell lines FU97, HGC-27, IM-95m, KATOIII, MKN-45, NUGC-4, OCUM-1, SNU-216, SNU-484, SNU-601, SNU-638 and SNU-719 were grown in RPMI-1640 medium, 10% fetal bovine serum (Sigma) and 1% penicillin–streptomycin (Invitrogen). Two hundred and ninety-three human embryonic kidney cells were grown in DMEM (high-glucose) medium, 10% fetal bovine serum (Sigma), 1 × non-essential amino acids (Invitrogen) and 1% penicillin–streptomycin (Invitrogen), and used for transcriptional reporter assays and lentivirus packaging. Antibodies The following antibodies were used for immunoblot analysis: ZAK TV-1 (Bethyl; A301-993A), ZAK TV-1 and TV-2 (Sigma; HPA017205), FLAG (Sigma; A8592), Tubulin (Sigma; T6074), and horseradish peroxidase-conjugated anti-mouse and anti-rabbit secondary antibodies (Jackson ImmunoResearch). The Sigma HPA017205 antibody also recognizes additional bands when probing for endogenous levels of ZAK, some of which run at the same molecular weight as ZAK TV-1. Therefore, the Bethyl A301-993A antibody was used for probing for endogenous ZAK TV-1. Lentivirus manipulation shRNAs were expressed in IM-95m, MKN-45 and SNU-216 cells using a lentiviral system. Three lentiviral shRNAs constructs targeting ZAK or a non-targeting control (NTC) were used in the study: pLKO.1-shNTC (Sigma; SHC002), pLKO.1 shZAK-1 (Sigma; TRCN0000003265), and pLKO.1-shZAK-2 (Sigma; TRCN0000003266). Briefly, 293 cells were transfected with pLKO.1-shRNA vector along with pCMV-VSVG and pCMV-dR8.9 to produce lentiviral particles. Viral particles were added to cells with 8 μg ml −1 polybrene and spin infected at room temperature (1,800 r.p.m., 30 min). Cells were selected 30 h after infection with 2 μg ml −1 puromycin. Transcriptional reporter assay ZAK transcript variant 1 (TV1) and 2 (TV2) were cloned into pCMV2a (Agilent Technologies) as BamHI/XhoI fragments. Transcriptional reporters were purchased from System Biosciences for AP1 (TR201PA-P), NFkB (TR012PA-P) and TCF/LEF (TR013PA-P). Two hundred and ninety-three cells were plated in 96-well format (15,000 cells per well) and plasmids were co-transfected with Fugene 6 (Promega). Reporter activation was measured after 48 h using the Dual-Glo luciferase system (Promega). Cell number was measured on a parallel plate using CellTiter-Glo (Promega). Accession codes: Sequencing and genotype data have been deposited in the European Genome-phenome Archive (EGA), which is hosted by the European Bioinformatics Institute (EBI), under the accession code EGAS00001000736. How to cite this article: Liu, J. et al. Integrated exome and transcriptome sequencing reveals ZAK isoform usage in gastric cancer. Nat. Commun. 5:3830 doi: 10.1038/ncomms4830 (2014).